Development of a high-throughput strategy for discovery of potent analogues of antibiotic lysocin E Lysocin E, a 37-membered natural depsipeptide, induces rapid bacteriolysis in methicillin-resistant Staphylococcus aureus via a unique menaquinone-dependent mechanism, presenting a promising therapeutic lead. Despite the great medical importance, exploring the potential utility of its derivatives as new platform structures for antibiotic development has remained a significant challenge. Here, we report a high-throughput strategy that enabled the preparation of thousands of analogues of lysocin E and large-scale structure-activity relationship analyses. We integrate 26-step total synthesis of 2401 cyclic peptides, tandem mass spectrometry-sequencing, and two microscale activity assays to identify 23 candidate compounds. Re-synthesis of these candidates shows that 11 of them ( A1 – A11 ) exhibit antimicrobial activity superior or comparable to that of lysocin E, and that lysocin E and A1 – A11 share l -Leu-6 and l -Ile-11. Therefore, the present strategy allows us to efficiently decipher biologically crucial residues and identify potentially useful agents for the treatment of infectious diseases. As the emergence of multidrug-resistant bacteria poses a serious threat to public health around the world [1] , [2] , [3] , as in the case with hospital-acquired methicillin-resistant Staphylococcus aureus (MRSA), there is an urgent need for the discovery and development of effective antibiotics with new modes of action against the resistant strains [4] , [5] . Natural products have been essential sources of new drugs for infectious diseases [6] , [7] , [8] , [9] . While having evolutionarily selected structures, natural products themselves do not necessarily provide optimal properties as therapeutic agents. To identify desirable drug candidates with enhanced antibacterial activity derived from a natural product, structure-activity relationship (SAR) studies are typically required through syntheses of a wide variety of analogues based on its structural framework [10] , [11] , [12] , [13] . Total synthesis offers the most flexible and powerful approach to generating diverse structures and therefore addresses major challenges in the SAR analysis, where structurally complex natural products are often difficult to isolate in large quantities or to chemically modify [14] . However, one-by-one multi-step synthesis of many analogues is extremely time-consuming and impractical. Consequently, the potential of natural products has not been fully explored due to lack of efficient and robust synthetic methods for analogue generation. A highly efficient strategy for preparing and evaluating the natural product-based compounds for the development of pharmaceuticals is therefore in high demand. Lysocin E ( 1 , Fig. 1a ) was isolated from Lysobacter sp. as a new antibiotic and structurally determined to be a 37-membered depsipeptide (molecular weight = 1618 Da) with an N-methylated amide and ester linkages [15] . The macrocyclic core of 12 residues contains four different non-proteinogenic d -amino acids ( d -Arg-2/7, N-Me- d -Phe-5, d -Gln-9, d -Trp-10) and is appended with ( R )-3-hydroxy-5-methylhexanamide. It displays potent activity against MRSA through rapid bacteriolysis with a minimum inhibitory concentration (MIC) of 4 μg/mL and a superior therapeutic effect in S. aureus -infected mice (ED 50 = 0.5 mg/kg) to that of vancomycin (ED 50 = 5.8 mg/kg) [15] . Our previous studies revealed that 1 exerts its activity by a mechanism distinct from any other antibiotics. It disrupts bacterial membrane through selective interaction with menaquinone (MK), which is essential for the respiration process driven by conversion between MK and its reduced form, menahydroquinone (MKH), in the cell membrane [16] , [17] . In vitro, 1 forms a 1:1 complex (K D = 4.5 μM) with menaquinone-4 (MK-4, 2 ), but has no affinity toward ubiquinone-10 (UQ-10, 3 ). Since ubiquinone is a coenzyme in the mammalian respiratory chain in mitochondria, the complexation selectivity of 1 is likely responsible for its selective toxicity against the bacteria. Recently, Walker et al. reported that 1 also interacts with lipid II [18] , a precursor for bacterial cell wall synthesis. The potent bactericidal activity and the novel mode of action make naturally occurring 1 a promising lead compound for the development of new antibiotics against multidrug-resistant bacteria. Fig. 1 Chemical structures of compounds used in this study. a Structures of lysocin E ( 1 ), menaquinone-4 (MK-4, 2 ), menahydroquinone-4 (MKH-4, 2 H ), and ubiquinone-10 (UQ-10, 3 ). Side-chain structures of 1 important for the potent antimicrobial activity are highlighted in orange (hydrophobic acyl chain), magenta (aromatic ring), and cyan (basic group). b Structure of the 1 -based one-bead-one-compound (OBOC) library comprising the bead-linked peptides. R 1-4 denote randomized side chains at residues-3, -6, -9, and -11 by split-and-mix synthesis. Table: Structures and properties of side chains at residues-3, -6, -9, and -11 of the bead-linked lysocin E analogues. One-letter codes of the amino acids and molecular weight of the residues are displayed in parentheses. The configurations of residues-3, -6, -9, and -11, sites for the bead-linking and macrolactamization, and direction of the chain elongation are also indicated. Hydrophobic, acidic, basic, hydroxy, primary amide, aromatic, and methyl groups are highlighted in orange, red, cyan, yellow, purple, magenta, and pink, respectively. TentaGel MB TentaGel Macrobeads. c Component amino acids for construction of the 1 -based OBOC library. Protective groups to be removed on a solid support are indicated in blue. Boc t -butoxycarbonyl; Fmoc 9-fluorenymethoxycarbonyl; Pbf 2,2,4,6,7-pentamethyldihydrobenzofuran-5-sulfonyl; TBS tert -butyldimethylsilyl; t -Bu tert -butyl; Tr triphenylmethyl Full size image The unique biological property of 1 prompted us to launch chemical and biological studies of 1 . In 2015, we achieved a full solid-phase total synthesis of 1 [19] . By taking advantage of the established synthetic strategy, we subsequently prepared 15 analogues with different side-chain structures [20] . This SAR study led us to dissect the key structural features (highlighted in color in Fig. 1a ) of 1 : (1) the cationic functionalities of d -Arg-2 and -7 for binding to the anionic polar heads of the membrane, (2) the hydrophobic acyl group at l -Thr-1 for partition into the membrane, and (3) the indole ring of d -Trp-10 and the phenyl ring of N-Me- d -Phe-5 for aromatic-aromatic interaction with MK [21] . However, none of the 15 analogues was more potent than the parent natural product 1 , exemplifying the formidable challenge in searching for more active analogues through one-by-one total synthesis. Here we report a high throughput platform for constructing and screening 2401 lysocin E analogues that had not been readily available en masse through total synthesis of individual compounds. It permits us to discover 18 hit compounds ( A1 – A18 ) with a hit rate of 0.7%, of which 11 compounds ( A1 – A11 ) are revealed to have antimicrobial activity more potent than or comparable to that of the parent natural product 1 , as well as high MK-dependent membrane lytic activity. Plan for construction of lysocin E-based OBOC library To find molecules with more potent antimicrobial activity, we envisioned to synthesize a much larger number of natural product analogues (>1000 molecules) than that used in conventional SAR studies of natural products [22] , [23] , [24] . To achieve high-throughput synthesis and evaluation of thousands of cyclic peptides, we adopted the one-bead-one-compound (OBOC) strategy (Fig. 1b ) [25] , [26] . Important features of this strategy are (i) the split-and-mix approach can readily diversify the structures, (ii) each bead displays a unique chemical entity, (iii) the chemical structure on a bead can be determined by tandem mass spectrometry (MS/MS) [27] , and (iv) both on-bead and in-solution assays can be used. Whereas the OBOC approach has provided a powerful tool for constructing a library of small peptides, it has not been applied to complex natural products except for in a few reports [28] , [29] . Nonetheless, we assumed that it would be possible to construct a 1 -based OBOC library because of the high efficiency of our synthetic route to 1 (Fig. 1c ) [19] , [20] . The full solid-phase synthesis of 1 was achieved in 8.0% total yield via stepwise elongation from the Wang resin-linked 7 using 4 – 6 and 8 – 14 , subsequent macrolactamization, and simultaneous acid-promoted removal of the protective groups ( t -Bu, Tr, Boc, TBS, Pbf [30] ) and the Wang resin. In designing the OBOC library of 1 with high hit rate, the sites of the structural alterations were selected so that the perturbation in the biologically important substructures and the overall synthetic efficiency would be minimized (Fig. 1a ). First, the C α -stereogenic centers of the 11 residues and the C α -methylene of Gly-4 were retained due to their potential influence on the bioactive three-dimensional conformation. Second, ( R )-3-hydroxy-5-methylhexanamide, d -Arg-2/7, N-Me- d -Phe-5, and d -Trp-10 were maintained, because their substitutions decreased the activities [20] . Third, l -Glu-8, and l -Thr-1/12 were not substituted. While l -Glu-8 is essential as an anchor to a solid support, a change in l -Thr-1/12 was presumed to affect the yield of the solid-phase esterification, which is generally more sensitive to the surrounding structures than an amidation. These considerations led us to determine l -Ser-3, l -Leu-6, d -Gln-9, and l -Ile-11 as the substitution sites for the library construction. As there was no prior knowledge on the structural requirements for residues-3, -6, -9, and -11 for improving activity, the side chains of substituting residues were diversified in terms of their physicochemical properties (Fig. 1b ). Hydrophobic (orange), acidic (red), basic (cyan), hydroxy (yellow), primary amide (purple), and aromatic (magenta) groups were selected for this purpose. As a chemical version of alanine-scanning mutagenesis [31] , substitution with the methyl group (pink) was also included. To achieve unambiguous structure determination of the compound on each bead by MS/MS analysis, each residue-n ( n = 3, 6, 9, 11) of the sequence must be identified with a unique molecular weight. As shown in Fig. 1b , the mass units of the side chains at residue-n (R 1-4 ) thus all differed. It should be noted that d -lysine was to be used as a basic substitution except for d -ornithine at residue-9, because d -glutamine (Mw = 128) as residue-9 of 1 , has the same mass number as d -lysine (Mw = 128). Thus, 12 amino acid components 15 – 26 were necessary for the library in addition to the 11 original components 4 – 14 contained in lysocin E (Fig. 1c ). Fig. 2 Synthesis and evaluation of bead-linked lysocin E. a Synthesis of bead-linked lysocin E 30 and establishment of the OBOC protocols. The fragmentation pattern of hydrolyzed 31 on MALDI-MS/MS is also shown. Reagents and conditions: a 20% piperidine/NMP, b HATU, HOAt, i -Pr 2 NEt, NMP, 40 °C (rt for 9 ). a.u. arbitrary unit, DIC N , N ’-diisopropylcarbodiimide, DMAP N , N -dimethyl-4-aminopyridine, HATU O -(7-aza-1 H -benzotriazol-1-yl)- N , N , N ’, N ’-tetramethyluronium hexafluorophosphate, HOAt 1-hydroxy-7-azabenzotriazole; HOBt 1-hydroxybenzotriazole; NMP N -methyl-2-pyrrolidone; PyBOP benzotriazol-1-yloxy)tripyrrolidinophosphonium hexafluorophosphate; TFA trifluoroacetic acid. b Color of 30 before ( 2 (−)) and after ( 2 (+)) incubation with 2 . c Color of the 3 beads of 2 (−) and 2 (+). Each bead is indicated by an arrow. d Growth inhibition of Staphylococcus aureus Smith ATCC 13709 caused by natural (0.04 μg per well, wells A and B) and 85% of single bead-derived 1 (wells C and D) in 10% BCS-doped Mueller Hinton Broth (40 μL) as growth medium. DMSO was used as vehicle control (wells E and F). Evaluation of the growth inhibitory activity was conducted as duplicate experiments. BCS bovine calf serum Full size image Randomization of the 4 positions with the 7 amino acid residues would generate the library comprising 2401 (=7 4 ) peptides. For the split-and-mix synthesis of the bead-linked peptides, TentaGel [32] beads were employed as a solid support (Fig. 1b ). The polyethyleneglycol (PEG) chains on TentaGel beads would facilitate efficient peptide elongation due to their high swelling property in organic solvents [33] , [34] , and reduce non-specific binding of hydrophobic molecules such as MK-4 ( 2 ). Furthermore, a high loading capacity (3.5 nmol per 0.3 mm bead) would provide sufficient sample quantity for the post-synthesis analyses. To maximize the coverage of this library without losing operational efficiency, the 3-fold number of beads (approximately 7510 beads) was to be included (expected coverage of the peptides = 95%) [35] . An o -nitroveratryl linker [36] , [37] was chosen on the basis of acid-stability and photocleavable property. The bead-linked peptides can be obtained upon acidic global deprotection, which are readily amenable for the on-bead complexation activity with 2 . Simple light-irradiation would liberate the peptides, which can be subjected to MS/MS sequencing and to the in-solution analysis of their antimicrobial activity. Synthesis and evaluation of bead-linked lysocin E Since one bead contains only less than 1 μg of a peptide, small-scale procedures should be devised prior to construction of the 1 -based OBOC library. Hence, we first aimed to synthesize the parent 1 using TentaGel beads to validate the feasibility of our OBOC strategy. Preparation of bead-linked 1 started with the conjugation of photocleavable linker 28 with the amine of TentaGel beads 27 (Fig. 2a ). The secondary alcohol of the linker was then condensed with the carboxylic acid of Fmoc-Glu-OAllyl 7 to afford 29 in 90% yield over 2 steps (3.2 nmol per bead). The thus-obtained beads were submitted to the Fmoc-based solid-phase peptide synthesis. Amide coupling was conducted at 40 °C under microwave-assisted conditions in NMP to facilitate the synthesis [38] , [39] . The linear dodecapeptide was elongated from 29 by 7 cycles of piperidine-promoted N α -deprotection and HOAt/HATU [40] -mediated amidation ( 4 – 6 , 9 , 11 , and 12 ), DIC/DMAP-promoted esterification ( 10 ), and then 3 cycles of N α -deprotection and amidation ( 8 , 13 , and 14 ). The Fmoc group of the N-terminus and the allyl group of the C-terminus of the product were then removed by treatment with piperidine, and subsequently with Pd(PPh 3 ) 4 and morpholine to provide the macrolactam precursor [41] . On-bead cyclization [42] was then effected using PyBOP/2,4,6-collidine [43] , leading to the 37-membered macrolactam. Finally, treatment of the macrolactam with aqueous TFA detached the side-chain protective groups to furnish the bead-linked lysocin E 30 . Despite its stability under acidic conditions, the linker of 30 was smoothly cleaved by dispersing in MeOH and irradiating ultra-violet light (365 nm), delivering the crude 1 . The overall yield from 29 to 1 over 26 steps was calculated to be 5.1% by MS and ultra-high-performance liquid chromatography (UHPLC) analyses (Supplementary Fig. 1 ), demonstrating that the efficiency of the procedure was comparable to that of the previous total synthesis (8.0%). Consequently, one bead after the synthesis contained 0.25 μg of 1 . Having optimized the synthesis of 1 for the OBOC format, we then needed to address the challenges in its structure determination by using only one bead. Sequencing of cyclic peptides is generally problematic, however, because of their complex fragmentation patterns caused by ring-opening at multiple positions [44] . Therefore, to simplify the analysis, the macrocycle of 1 was linearized by exploiting the single ester linkage between l -Thr-1 and -12. Specifically, 1 was treated with 1% NH 3 in MeOH/H 2 O to generate the linear seco acid 31 . Matrix-assisted laser desorption/ionization (MALDI) MS/MS spectrometry of 31 afforded high-quality fragment ions, matching to the amino-acid sequence of 1 . Because of its high sensitivity, the MS/MS sequencing analysis required only 15% of 1 on one bead (0.04 μg). Next, the feasibility of the on-bead complexation assay was assessed using bead-linked lysocin E 30 and MK-4 ( 2 ). Our initial assay based on the finding that 1 and 2 form a red precipitate upon complexation (Supplementary Fig. 2 ) was not robust [45] , because the magnitude of the red color was not proportional to the amount of captured 2 (Fig. 2b, c ). We therefore developed a fluorescence-based method for quantifying 2 by reducing its naphthoquinone moiety to fluorescent hydroquinone 2H . One bead of 30 was incubated with 2 in MeOH, washed by MeOH in a microplate well, and then the bead-bound 2 was eluted under more forcing hydrophobic conditions ( n -BuOH at 50 °C). The eluate containing 2 was treated with NaBH 4 in n -BuOH to produce 2H [46] . The fluorescence intensity of 2H was evaluated to determine the quantity of 2 bound to one bead of 30 . The method was found with a small margin of error (1026 ± 64 a.u. ), indicating its high accuracy (Fig. 2a and Supplementary Fig. 3 ). Importantly, the structure of 1 remained intact during the complexation assay as judged by UHPLC and mass analyses. Finally, a microscale antimicrobial assay was developed to evaluate the activity of 1 in solution phase. Since MS/MS-sequencing consumed 15% of the single-bead-derived 1 , only 0.21 μg of 1 corresponding to remaining 85% of the sample could be applied to the assay. The original MIC value (2–4 μg/mL) of 1 against S. aureus was, however, too high to reliably detect its activity in a submicrogram scale. Since 1 has potent therapeutic effects in S. aureus -infected mice (ED 50 = 0.5 mg/kg), we assumed that mimicking the in vivo conditions would lower the MIC value of 1 . 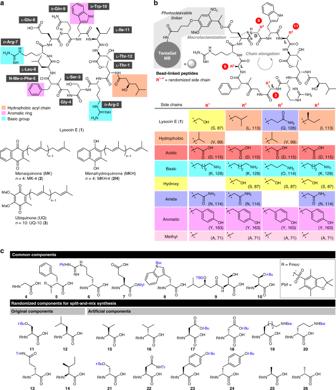Fig. 1 Chemical structures of compounds used in this study.aStructures of lysocin E (1), menaquinone-4 (MK-4,2), menahydroquinone-4 (MKH-4,2 H), and ubiquinone-10 (UQ-10,3). Side-chain structures of1important for the potent antimicrobial activity are highlighted in orange (hydrophobic acyl chain), magenta (aromatic ring), and cyan (basic group).bStructure of the1-based one-bead-one-compound (OBOC) library comprising the bead-linked peptides. R1-4denote randomized side chains at residues-3, -6, -9, and -11 by split-and-mix synthesis. Table: Structures and properties of side chains at residues-3, -6, -9, and -11 of the bead-linked lysocin E analogues. One-letter codes of the amino acids and molecular weight of the residues are displayed in parentheses. The configurations of residues-3, -6, -9, and -11, sites for the bead-linking and macrolactamization, and direction of the chain elongation are also indicated. Hydrophobic, acidic, basic, hydroxy, primary amide, aromatic, and methyl groups are highlighted in orange, red, cyan, yellow, purple, magenta, and pink, respectively. TentaGel MB TentaGel Macrobeads.cComponent amino acids for construction of the1-based OBOC library. Protective groups to be removed on a solid support are indicated in blue. Boct-butoxycarbonyl; Fmoc 9-fluorenymethoxycarbonyl; Pbf 2,2,4,6,7-pentamethyldihydrobenzofuran-5-sulfonyl; TBStert-butyldimethylsilyl;t-Butert-butyl; Tr triphenylmethyl Screening of the additives indeed revealed that bovine calf serum (BCS) dramatically enhanced the antimicrobial activity of 1 (Supplementary Table 1 ), although the factors responsible for this remarkable effect remain to be identified. Specifically, the MIC values of 1 against methicillin-susceptible S. aureus (MSSA1) and S. aureus Smith ATCC 13709 were decreased by 64-fold (0.0625 μg/mL) by adding 10% BCS to the growth medium. By applying these conditions (Fig. 2d ), both natural product 1 (0.04 μg, wells A and B) and single-bead-derived 1 (corresponding to 85% of the cleaved peptide sample, wells C and D) were shown to completely inhibit the growth of S. aureus , whereas no growth inhibition was observed in the control wells (E and F). Taken together, these established experimental protocols enabled synthesis, structural determination, and functional evaluation by using 1 derived from a single bead. Construction of the lysocin E-based OBOC library Having successfully completed the pilot study using 1 , the high throughput scheme for the full-scale OBOC library was planned as shown in Fig. 3 . First, the bead-linked 2401 peptides are to be generated by parallel solid-phase syntheses using the split-and-mix approach. Second, 2 -complexation activity is assessed by a fluorescence-based assay for all the beads in a parallel format in the microplate wells. Third, upon photocleavage, 15% aliquot of the single-bead derived peptide is linearized to determine its sequence by MS/MS analysis. Fourth, the remaining 85% aliquot is evaluated for the antimicrobial activity. To facilitate an efficient screening process, only the positive compounds in the second step were to be used for the third and fourth steps. We envisaged that the combined use of on-bead and in-solution assay systems would lead to the rapid discovery of biologically active analogues of 1 that share the 2 -dependent mechanism of action. Fig. 3 Overview of the OBOC strategy. A high throughput platform for constructing and screening 2401 lysocin E analogues is shown Full size image The OBOC library comprising 2401 peptides was constructed by applying split-and-mix methods at residues-3, -6, -9, and -11 (Fig. 4a ). The reagents and conditions for amidation, esterification, macrocyclization, and deprotection were the same as those established in Fig. 2a , while 12 components 15 – 26 were additionally employed for the randomization. Thus, 7 -conjugated 29 consisting of 7510 beads was transformed into N α -Fmoc protected dipeptide 32 in 2 steps. In the first randomization step at residue-6, the beads of 32 were divided into 7 pools, which were separately deprotected and condensed with the original ( 12 ) and 6 different Fmoc amino acids ( 11 , 17 , 19 , 22 , 23 , and 25 ). Then, all the beads were mixed again and subjected to stepwise chain extension using 5 and 4 to afford pentapeptide 33 containing 7 structures. The second split-and-mix synthesis at residue-3 using the 7 components ( 11 , 15 , 17 , 19 , 22 , 23 , and 25 ) was followed by one-by-one N α -deprotection/condensation of 6 , 9 , and 10 , giving rise to nonapeptide 34 (49 structures). Further attachment of the 3 amino acid residues included randomization at residues-11 and -9 and simple extension at residue-10, leading to linear dodecapeptide 36 (2401 structures). Finally, 36 was collectively converted into the bead-linked 2401 cyclic peptides via sequential base-promoted removal of the Fmoc group, palladium-mediated removal of the allyl group, 37-membered ring cyclization, and on-bead global deprotection. The overall yields of the peptides were assumed to be approximately 2%–12% (0.1–0.6 μg of a peptide per bead) according to the yield of 1 in Fig. 2a and the yields of the re-synthesized compounds in Table 1 , although calculation of the precise yields was not feasible at this stage. Fig. 4 Synthesis and screening of the OBOC library. a Synthesis of 1 -based OBOC library comprising 2401 bead-linked peptides. Reagents and conditions: a 20% piperidine/NMP, b HATU, HOAt, i -Pr 2 NEt, NMP, 40 °C (rt for 9 ). b Schematic diagram of selection of the compounds belonging to groups A–C. A dot plot of fluorescence intensity against bead number (1–7510) in the 2 -complexation assay is also displayed. Fluorescence intensity corresponds to the relative amount of 2H . 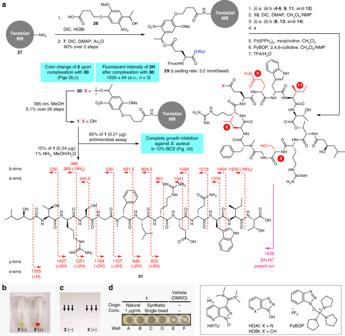Fig. 2 Synthesis and evaluation of bead-linked lysocin E.aSynthesis of bead-linked lysocin E30and establishment of the OBOC protocols. The fragmentation pattern of hydrolyzed31on MALDI-MS/MS is also shown. Reagents and conditions: a 20% piperidine/NMP, b HATU, HOAt,i-Pr2NEt, NMP, 40 °C (rt for9). a.u. arbitrary unit, DICN,N’-diisopropylcarbodiimide, DMAPN,N-dimethyl-4-aminopyridine, HATUO-(7-aza-1H-benzotriazol-1-yl)-N,N,N’,N’-tetramethyluronium hexafluorophosphate, HOAt 1-hydroxy-7-azabenzotriazole; HOBt 1-hydroxybenzotriazole; NMPN-methyl-2-pyrrolidone; PyBOP benzotriazol-1-yloxy)tripyrrolidinophosphonium hexafluorophosphate; TFA trifluoroacetic acid.bColor of30before (2(−)) and after (2(+)) incubation with2.cColor of the 3 beads of2(−) and2(+). Each bead is indicated by an arrow.dGrowth inhibition ofStaphylococcus aureusSmith ATCC 13709 caused by natural (0.04 μg per well, wells A and B) and 85% of single bead-derived1(wells C and D) in 10% BCS-doped Mueller Hinton Broth (40 μL) as growth medium. DMSO was used as vehicle control (wells E and F). Evaluation of the growth inhibitory activity was conducted as duplicate experiments. BCS bovine calf serum Beads exhibiting a fluorescence intensity >1000 a.u. are plotted as red dots. Source data are provided as a Source Data file Full size image Table 1 Structures and activities of lysocin E and 32 analogues Full size table MK-4–complexation assay and MS/MS-sequencing An on-bead MK-4 ( 2 )–complexation assay using the 7510 beads revealed significantly varied activities (Fig. 4b ). Based on the fluorescence intensity of 1026 ± 64 a.u. for 30 carrying the parent lysocin E structure, we defined the 241 beads exhibiting fluorescence intensities of >1000 a.u. (Fig. 4b , red dots) as the hit beads. Approximately top 3% of the entire beads was selected for the subsequent experiments. Next, the structures of the 241 bead-linked peptides were determined. After releasing the cyclic peptides from the beads by photocleavage, the 15% fraction of each peptide was chemoselectively hydrolyzed to produce the linear peptide. MALDI-MS/MS analysis of 241 linear dodecapeptides showed that 237 afforded clear parent ions and fragmentation patterns, permitting us to unambiguously establish their structures (Supplementary Tables 2 – 4 ). As a result, 166 unique structures were identified. Importantly, one of the 166 compounds turned out to be the parent 1 , demonstrating the reliability of the split-and-mix synthesis of thousands of peptides and the validity of the 2 -complexation assay for selecting the active molecules from the mixture. Finally, the 166 positive compounds identified in the on-bead assay were evaluated in an in-solution antimicrobial assay. We found that 23 compounds including 1 completely suppressed the growth of S. aureus Smith ATCC 13709 in 10% BCS-supplemented medium (Supplementary Fig. 4 and Supplementary Tables 2 – 4 ). For further analyses, we designated 22 compounds that were positive in the two assays as A1 – A22 (group A), and 10 peptides positive in the first assay and negative in the second assay as B1 – B5 (group B) and C1 – C5 (group C). B1 – B5 correspond to the top 5 compounds in the 2 -complexation assay and C1 – C5 were randomly selected from the remaining compounds. Antimicrobial spectra and membrane-disrupting activity To validate the OBOC strategy and evaluate the detailed biological activities, the 32 analogues of 1 ( A1 – A22 , B1 – B5 , and C1 – C5 ) were individually re-synthesized in several milligram scales according to the original solid-phase synthetic route to 1 [19] , [20] . The crude materials were purified by HPLC to generate A1 – A22 , B1 – B5 , and C1 – C5 in 1.8–12% total yield over 25 steps (Supplementary Tables 5 and 6 ). The total syntheses of the 32 structurally complex analogues in consistent overall yields (5.6 ± 3.0%) corroborated the robustness and generality of the full-solid phase synthetic route. The antimicrobial activities of the fully synthetic 32 analogues were evaluated and compared with those of 1 (Table 1 ). The MIC values were determined by the 2-fold serial dilution procedure against 6 strains of Gram-positive bacteria. In addition, effects of the peptides against MSSA1 were evaluated in the absence or presence of BCS. The compounds in each group A, B, or C are listed in descending order of the activity against MSSA1 in the presence of 10% BCS. When the compounds displayed the same MIC values toward the BCS-supplemented MSSA1, the values for the BCS-unsupplemented MSSA1 were used for their ordering. Most significantly, the MIC values of the 11 analogues A1 – A11 against MSSA1 were found to be 0.015–0.0625 μg/mL upon addition of 10% BCS to the growth medium, thus having activities more potent than or equipotent to that of 1 (0.0625 μg/mL). Among them, the 3 analogues, A1 , A2 , and A3 , showed 4-fold higher antimicrobial activities than the parent natural product 1 . Similarly to 1 (0.25 μg/mL), A1 – A3 also displayed high activities against BCS-supplemented MRSA4 (0.25, 0.25, and 0.125 μg/mL, respectively), suggesting their potential utility in the treatment of MRSA infections. 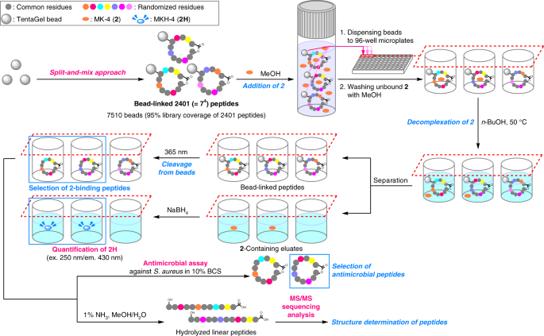Fig. 3 Overview of the OBOC strategy. A high throughput platform for constructing and screening 2401 lysocin E analogues is shown In addition, the 7 compounds A12 – A18 retained strong antimicrobial effects although somewhat weaker than 1 . On the other hand, the remaining 4 peptides, A19 – A22 , in group A have MIC values comparable to or higher than 6.7 ± 3.7 μg/mL, which was the upper threshold of the one-bead antimicrobial assay calculated from the molecular weights and the overall yields of the resynthesized 33 peptides. These false-positive compounds could be selected because of active impurities generated during the split-and-mix synthesis. Consistent with the high-throughput in-solution antimicrobial assay (Fig. 4b ), none of the compounds in groups B ( B1 – B5 ) and C ( C1 – C5 ) had the low MIC values. The results that 83% of 23 peptides in group A and 0% of 10 peptides in groups B and C were active therefore validated our screening system for the discovery of multiple active analogues. We also assessed the antimicrobial activity of the 33 compounds in groups A–C against the 6 Gram-positive bacteria in the absence of BCS. Natural product 1 and 18 analogues A1 – A18 were active against all the strains including MRSA4, whereas A19 – A22 , B1 – B5 , and C1 – C5 had only weak or negligible effects on the bacteria. Intriguingly, while BCS enhanced the activities of A1 – A14 toward MSSA1 by 16 to 533 times, the additive only increased the activities of A15 – A18 by 2–4 fold. The strain selectivity of A1 – A18 was found to be similar. They are more active toward S. haemolyticus and B. cereus , and less active toward L. monocytogenes . A15 and A17 were slightly different from the other peptides, however, having only weak effects on L. monocytogenes (MIC = 64 μg/mL), and on B. cereus and B. subtilis (MIC = 16 μg/mL), respectively. These results demonstrated that structural alternations of 1 are effective in attenuating the strain selectivity. To confirm that the synthetic analogues share the mode of action of 1 , we quantified the MK-4 ( 2 )-dependent membrane lytic activity of the 33 synthetic peptides as EC 50 values by employing liposomes as bacterial cell membrane models [47] . Large unilamellar vesicles (LUVs) comprising egg yolk phosphatidylcholine (PC)/egg yolk phosphatidylglycerol (PG) (50:50 ratio) were prepared to mimic the negatively charged surface of bacterial membranes [48] . The PC/PG LUVs were doped with 1.25 mol% of MK-4 ( 2 ) [49] , [50] , or with 1.25 mol% of UQ-10 ( 3 ) to assess the selectivity toward 2 over 3 . The EC 50 values of 1 for disrupting PC/PG/ 2 , PC/PG/ 3 , and PC/PG LUVs were determined to be 19.5 nM, 92.0 nM, and 559 nM, respectively (Table 1 ), confirming the 2 -dependent lysis by 1 . The selectivity index of 1 toward 2 over 3 was calculated to be 4.7 (=92.0/19.5). Remarkably, 25 of the 32 analogues ( A1 – A20 , B1 , B3 , and C1 – C3 ) had detectable EC 50 values for the PC/PG/ 2 LUVs and selectivity indexes greater than 2.7. Importantly, the 11 most potent antimicrobial compounds A1 – A11 displayed membrane-disrupting activities against the PC/PG/ 2 LUVs (EC 50 = 10.7–38.8 nM) comparable to that of 1 (19.5 nM). Thus, it is expected that 1 and A1 – A11 share the same 2 -dependent mechanism of action. It is also noteworthy that the selectivity indexes of A7 (19.7), A14 (>19.7), and A16 (20.6) were higher than that of 1 (4.7), demonstrating that the 2 -selectivity can be enhanced by structural alteration of 1 . These data together allowed us to gather valuable information on the structural requirements for the antimicrobial and 2 -selective membrane-disrupting activities (Fig. 5a ). The most remarkable finding is that leucine (L) at residues-6 and isoleucine (I) at residue-11 are both shared among the parent 1 , all the 11 potent analogues A1 – A11 and the less active A12 – A18 except for A15 . Thus, these residues are most likely to be essential for the potent antimicrobial functions. As leucine and isoleucine are hydrophobic and bulky, their side chains can interact with hydrophobic tails of bacterial membrane lipids or 2 , and/or organize the bioactive conformation of the peptides [51] . In contrast to the conserved residues-6 and -11, residues-3 and -9 are significantly varied, indicating the less stringent requirement for these substructures for the activity. A1 – A3 with the highest antimicrobial activities possess alanine (A) or lysine (K) at residue-3 and valine (V) or glutamine (Q) at residue-9. For A7 , A14 , and A16 with the highest 2 -selectivity, residue-9 is substituted with ornithine (O), implying that ornithine may play specific roles to augment the activity. It is interesting to note that the only difference between the most potent analogue A1 and 1 is the presence or absence of the hydroxy group at residue-3. A15 is different from 1 at residues-3 (alanine), -9 (tyrosine), and -11 (tyrosine) (Fig. 5b ), suggesting this unique sequence is responsible for insensitivity to the BCS-addition and different bacterial strain selectivity. Since changing the leucine (L) at residue-6 of A15 to alanine (A) gives inactive analogue C2 , it confirms the significance of l -Leu-6 for the activity. Overall, the present strategy proved to be effective for deciphering the crucial structural factors for enhancing and modulating the functions of 1 . Fig. 5 Structures of lysocin E and 19 analogues. a Structures of 1 and its antimicrobial analogues A1 – A14 and A16 – A18 . b Structures of antimicrobial analogue A15 and non-antimicrobial analogue C2 Full size image We discovered 18 antimicrobial analogues A1 – A18 of complex peptide natural product 1 by developing a high throughput method that integrates 26-step solid-phase total synthesis of 2401 cyclic peptides, MS/MS-sequencing, and two different microscale activity assays. Our design strategy for the peptide library involved three criteria. Four amino acid residues of 1 (residues-3, -6, -9, and -11) were chosen as the site of randomization based on the previous SAR data and the synthetic efficiency. The 7 amino-acid components were employed to substitute the sites of randomization in order to explore diverse structures in the library with varying physicochemical properties and to represent unique molecular weight for unambiguous structure determination by MS/MS. The split-and-mix synthesis was achieved in a submicrogram scale to generated the 2401 cyclic peptides on TentaGel beads with a photocleavable linker. The on-bead complexation assay with 2 and MS/MS-sequencing of photocleaved and linearized peptides identified 166 distinct sequences. Based on their in-solution assay against MSSA1 in the presence of BCS, they were further classified into antimicrobial ( 1 and A1 – A22 , 23 compounds) and non-antimicrobial groups (143 compounds). To validate the results obtained by the OBOC-based high throughput approach, active analogues A1 – A22 , and inactive analogues B1 – B5 (top 5 of the first assay) and C1 – C5 (random extraction) were all re-synthesized in a milligram scale. Among them, 18 compounds, A1 – A18 , proved to be active against MSSA1 under the BCS-supplemented conditions, demonstrating the high fidelity and high hit-rate (0.7%) of the developed screening system. Remarkably, A1 – A3 had 4-fold higher and comparable effects toward MSSA1 and MRSA4, respectively, indicating their potential superiority to 1 as antibiotic agents. More active A1 – A3 and comparably active A4 – A11 also exhibited antimicrobial effects against 6 Gram-positive bacteria with selectivity profiles similar to that of 1 and share the 2 -dependent membrane-disrupting functions. The key common structural elements for A1 – A18 except for A15 were l -leucine at residue-6 and l -isoleucine at residue-11, revealing, for the first time, the significance of these hydrophobic amino acids. This SAR studies on a high number of lysocin E analogues provided large data sets that were previously unavailable, and led us to identify potentially superior agents for the treatment of infectious diseases caused by Gram-positive bacteria, including MRSA. Improving the activities of architecturally complex natural products is extremely challenging often due to lack of SAR information and synthetic accessibility. Thus, the discovery of the more potent synthetic analogues A1 – A3 , in particular, highlights the advantage of the present OBOC approach over the conventional one-by-one synthesis or rational design approach. As an OBOC library is extremely useful for rapid exploration of the biologically relevant chemical space around natural products, the overall methodology developed, here will be widely applicable as a promising strategy for extracting key structural features and identifying more biologically active analogues of natural products beyond this study. General remarks All reactions sensitive to air and/or moisture were carried out under argon (Ar) atmosphere in dry solvents, unless otherwise noted. CH 2 Cl 2 , DMF, and Et 2 O were purified by a Glass Contour solvent dispensing system (Nikko Hansen). All other reagents were used as supplied unless otherwise stated. Solid-phase peptide synthesis (SPPS) was performed on a microwave-assisted peptide synthesizer MWS-1000 (EYELA) using a sealed reaction vessel, a reaction temperature of which was monitored by an internal temperature probe. Optical rotations were recorded on a P-2200 polarimeter (JASCO). Infrared (IR) spectra were recorded on an FT/IR-4100 spectrometer (JASCO) as a thin film on a CaF 2 . 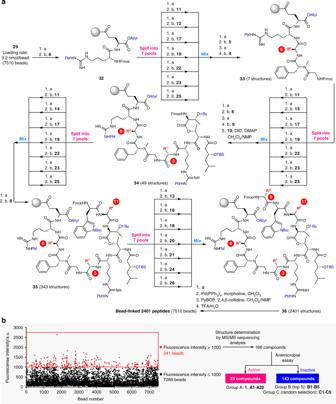Fig. 4 Synthesis and screening of the OBOC library.aSynthesis of1-based OBOC library comprising 2401 bead-linked peptides. Reagents and conditions: a 20% piperidine/NMP, b HATU, HOAt,i-Pr2NEt, NMP, 40 °C (rt for9).bSchematic diagram of selection of the compounds belonging to groups A–C. A dot plot of fluorescence intensity against bead number (1–7510) in the2-complexation assay is also displayed. Fluorescence intensity corresponds to the relative amount of2H. Beads exhibiting a fluorescence intensity >1000 a.u. are plotted as red dots. Source data are provided as a Source Data file 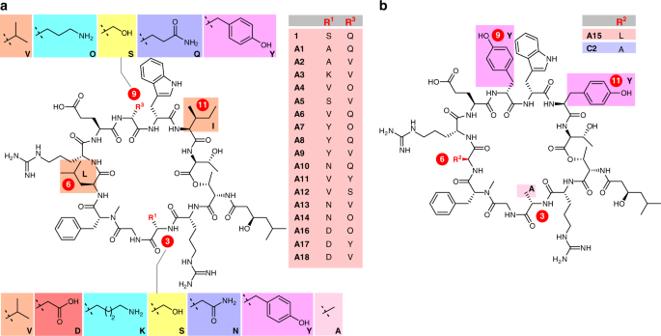Fig. 5 Structures of lysocin E and 19 analogues.aStructures of1and its antimicrobial analoguesA1–A14andA16–A18.bStructures of antimicrobial analogueA15and non-antimicrobial analogueC2 1 H and 13 C NMR spectra were recorded on an ECX 500 (500 MHz for 1 H NMR) spectrometer, an ECZ 500 R (500 MHz for 1 H NMR) spectrometer (JEOL), or an Avance III HD 800 MHz equipped with CryoProbe (800 MHz for 1 H NMR, 200 MHz for 13 C NMR) (Bruker). Chemical shifts are denoted in δ (ppm) relative to residual solvent peaks as internal standard (DMSO- d 6 , 1 H δ 2.50, 13 C δ 39.5). HRMS spectra were recorded on a MicrOTOFII (Bruker Daltonics) electrospray ionization time-of-flight (ESI-TOF) mass spectrometer. UV absorbance was measured on a UV-1800 UV-VIS spectrophotometer (Shimadzu). High performance liquid chromatography (HPLC) experiments were performed on a HPLC system equipped with a PU-2089 Plus intelligent pump or a HPLC system equipped with a PU-2086 Plus intelligent pump (JASCO). Ultrahigh-performance liquid chromatography (UHPLC) experiments were performed on a X-LC system (JASCO). Experimental data For MS/MS spectra of compounds A1 – A22 , B1 – B5 , and C1 – C5 , see Supplementary Figs. 10 – 42 . For 1 H, 13 C NMR, 1 H– 1 H DQF-COSY, 1 H– 1 H TOCSY, 1 H– 1 H NOESY, 1 H– 13 C HMBC, and 1 H– 13 C HSQC of A1 – A3 , see Supplementary Figs. 43 – 54 . For chemical shifts of compounds A1 – A3 , see Supplementary Tables 5 and 6 . For 1 H NMR spectra of compounds A4 – A22 , B1 – B5 , and C1 – C5 , see Supplementary Figs. 55 – 69 . For HPLC charts for purification of synthetic peptides, see Supplementary Figs. 70 – 134 . For UHPLC charts for purified synthetic peptides, see Supplementary Figs. 135 – 172 . For MS spectra of 241 bead-derived linear peptides, see Supplementary Figs. 173 – 213 . For the experimental procedures and spectroscopic data of compounds, see Supplementary Methods . Reporting summary Further information on research design is available in the Nature Research Reporting Summary linked to this article.